In vivoimaging of virological synapses Retroviruses such as the human immunodeficiency virus, human T-cell lymphotropic virus and murine leukaemia virus are believed to spread via sites of cell–cell contact designated virological synapses. Support for this model is based on in vitro evidence in which infected cells are observed to specifically establish long-lived cell–cell contact with uninfected cells. Whether virological synapses exist in vivo is unknown. Here we apply intravital microscopy to identify a subpopulation of B cells infected with the Friend murine leukaemia virus that form virological synapses with uninfected leucocytes in the lymph node of living mice. In vivo virological synapses are, like their in vitro counterpart, dependent on the expression of the viral envelope glycoprotein and are characterized by a prolonged polarization of viral capsid to the cell–cell interface. Our results validate the concept of virological synapses and introduce intravital imaging as a tool to visualize retroviral spreading directly in living mice. Retroviruses such as the human immunodeficiency virus (HIV-1), human T-cell lymphotropic virus and murine leukaemia virus (MuLV) have been observed in vitro to spread from infected to uninfected cells via long-lived cell–cell contacts [1] , [2] , [3] , [4] , [5] . Based on their resemblance to immunological synapses found between antigen-presenting cells and T lymphocytes, these structures were designated virological synapses [1] , [2] , [3] . Virological synapses are the consequence of interactions between the viral envelope (Env) glycoproteins expressed in the infected cells and receptor in the target cells [3] , [4] , [6] , [7] . The accumulation of Env and receptor at the cell–cell interface subsequently draws viral particles to the synapse for subsequent transmission [3] , [4] , [5] , [8] . In vitro adhesive interactions between infected and uninfected cells can exhibit different morphologies, from broad long-lived cell–cell contacts [3] , [5] , [8] , [9] and thin filopodial/nanotubular interactions [4] , [10] to more loose and transient interactions [11] , [12] . Polysynapses, cell–cell contacts between a single donor and multiple target cells have also been observed [6] . Whether long-lived virological synapses exist in vivo has remained unknown. Here we have applied a visual approach to ask whether any specific cell types infected with Friend-MuLV (F-MuLV) can form structures in vivo with uninfected cells that resemble in vitro virological synapses. To visualize retrovirus-infected cells in vivo , we have established intravital microscopy of F-MuLV-infected lymphocytes in the lymph node of living mice. F-MuLV infects many cell types expressing the receptor mCAT-1 and causes viremia in mice [13] . At late stages of infection, recombination events with endogenous viruses lead to the rise of pathogenic viruses that cause erythroleukemia [13] . The early steps in the spreading of the original replication-competent F-MuLV are poorly understood. Here we identify infected B cells in vivo that engage in long-lived interactions with neighbouring uninfected cells depending on an interaction between the viral Env glycoprotein and its cellular receptor mCAT-1. Infected B cells specifically interact with uninfected CD4 + T cells and CD19 + B cells in vitro and their ability to interact correlates with the spread of the viral infection in mice. Our data suggest that virological synapses exist in vivo and likely contribute to the spread of viral infections in living organisms. Intravital microscopy identifies immobile infected B cells To identify a cell type capable of forming virological synapses to promote viral spread in vivo , we established adoptive transfer protocols that allowed the monitoring of infected lymphocytes within the lymph node of mice. Briefly, primary mouse T and B lymphocytes were prepared from transgenic mice expressing cytoplasmic red fluorescent protein (RFP) and infected ex vivo with F-MuLV generating green fluorescent protein (GFP)-labelled viral particles (F-MuLV Gag-GFP). These lymphocytes generate fluorescently labelled viral particles that can be released and transmitted to neighbouring cells, but cannot spread as they lack Pol. Lymphocytes were adoptively transferred subcutaneously (s.c.) into C57BL/6 mice to visualize uninfected (red) and F-MuLV-infected (red/green) cells within the popliteal lymph node ( Supplementary Fig. S1 ). Infected T cells were migratory and did not exhibit an immobile cell population as would be expected from cells forming virological synapses (data not shown). Interestingly, infected B cells, while only insignificantly reduced in their average migration speed, featured an elevated number of immobile cells ( Fig. 1a ; Supplementary Movies 1 and 2 ). To specifically ask whether this immobile B cell population is influenced by the expression of the viral Env glycoprotein, we compared the behaviour of F-MuLV-infected B cells expressing wild-type (WT) Env with that of infected B cells lacking Env. Strikingly, the percentage of cells in each experiment migrating <2 μm min −1 , generally defined as a stop in migration for lymphocytes in vivo [14] , was significantly increased for F-MuLV-infected B cells expressing WT Env protein (WT, 26%) as compared with cells lacking Env (ΔEnv, 7%; Fig. 1c ). The arrest coefficient was more than threefold elevated in cells expressing Env (WT, 15%) as compared with cells lacking Env (ΔEnv, 4%) confirming the Env dependence of the static nature of these infected B cells ( Fig. 1d ). The comparison of B cells infected by F-MuLV containing or lacking Env is most informative. Some B cells with undetectably low Gag-GFP expression may still express low levels of Env that would lower the migration speed of the ‘uninfected’ B-cell population and so explain the intermediate phenotype. 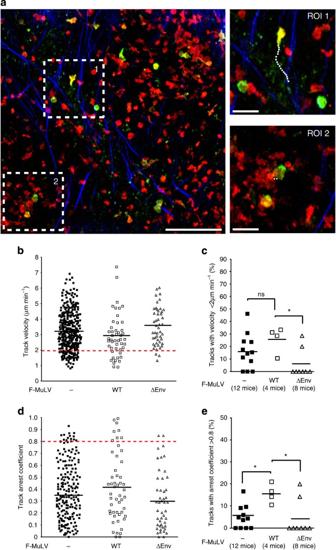Figure 1: Intravital microscopy of F-MuLV-infected B cells. (a) Intravital microscopy images of B cells (red) infected with F-MuLV Gag-GFP (green) within the popliteal lymph node of living C57BL/6 mice. Collagen fibres are shown in blue. Region of interest (ROI) 1 shows the track of a migrating Gag-GFP-positive B cell >20 min. ROI 2 displays two static infected B cells. White dots demonstrate the movement >20 min. The corresponding time-lapse movie isSupplementary Movie 1. Scale bar, 100 μm in overview image and 20 μm in images of ROI 1, 2. (b) Track velocity of uninfected (290 tracks, 12 mice) and infected B cells containing WT Env (WT, 48 tracks, 4 mice) or lacking Env (ΔEnv, 48 tracks, 8 mice). (c) Percentage of the static cell population (<2 μm min−1) as shown below the red line inbfor each independent experiment. Not infected compared with WT:ns (nonsignificant)P=0.1619; WT compared with ΔEnv: *P=0.0182 (Mann–Whitney test). (d) Arrest coefficient of tracks described inb. (e) Percentage of the static cell population that remained arrested (<2 μm min−1) >80% of imaging time above red line indfor each independent experiment. Not infected compared with WT: *P=0.0122; WT compared with ΔEnv: *P=0.0457 (Mann–Whitney test). Figure 1: Intravital microscopy of F-MuLV-infected B cells. ( a ) Intravital microscopy images of B cells (red) infected with F-MuLV Gag-GFP (green) within the popliteal lymph node of living C57BL/6 mice. Collagen fibres are shown in blue. Region of interest (ROI) 1 shows the track of a migrating Gag-GFP-positive B cell >20 min. ROI 2 displays two static infected B cells. White dots demonstrate the movement >20 min. The corresponding time-lapse movie is Supplementary Movie 1 . Scale bar, 100 μm in overview image and 20 μm in images of ROI 1, 2. ( b ) Track velocity of uninfected (290 tracks, 12 mice) and infected B cells containing WT Env (WT, 48 tracks, 4 mice) or lacking Env (ΔEnv, 48 tracks, 8 mice). ( c ) Percentage of the static cell population (<2 μm min −1 ) as shown below the red line in b for each independent experiment. Not infected compared with WT: ns (nonsignificant) P =0.1619; WT compared with ΔEnv: * P =0.0182 (Mann–Whitney test). ( d ) Arrest coefficient of tracks described in b . ( e ) Percentage of the static cell population that remained arrested (<2 μm min −1 ) >80% of imaging time above red line in d for each independent experiment. Not infected compared with WT: * P =0.0122; WT compared with ΔEnv: * P =0.0457 (Mann–Whitney test). Full size image F-MuLV-infected B cells form virological synapses in vivo F-MuLV virological synapses observed in vitro are characterized by an Env-dependent polarization of Gag to the cell–cell interface [8] . We therefore analysed the subcellular distribution of F-MuLV Gag-GFP (green) in vivo in static B cells (red) expressing or lacking Env. To this end, we quantified the GFP fluorescence at the cell surface by defining the cell shape using cytoplasmic RFP and displayed the GFP intensity as a 0–360° line profile ( Fig. 2a ). This analysis revealed a striking polarization of Gag in Env-expressing cells ( Fig. 2b , Supplementary Movies 3 and 4 ). Env-dependent Gag polarization towards one side frequently remained stable for the duration of the imaging time of ~25–60 min ( Fig. 2b for a period of 15 min, Supplementary Movie 3 ). To compare the distribution of Gag in static B cells expressing or lacking F-MuLV Env, we prepared an average polarization profile for individual cells over time ( Fig. 2c ). Analysing multiple static B cells confirmed the strict Env-dependent polarization of Gag ( Fig. 2d ). A Gag polarization coefficient defined to describe the extent of Gag polarization in terms of intensity, width and duration ( Supplementary Fig. S2 ) was fivefold enhanced in cells infected with F-MuLV expressing Env as compared with F-MuLV lacking Env ( Fig. 2e ). Importantly, F-MuLV Env carrying a point mutation in the receptor-binding domain (EnvS84I) [4] behaved identical to F-MuLV lacking Env, demonstrating that the polarization of Gag was the consequence of an Env-receptor-induced virological synapse ( Fig. 2d ). The strong prolonged Gag polarization was also apparent from a heat map display of Gag fluorescence intensity along the plasma membrane (0–360°) over time ( Fig. 2f ). Also, besides a predominance of single virological synapses, polysynapses as well as thin membrane contacts carrying F-MuLV Gag-GFP, previously reported in vitro for HIV and MLV [4] , [6] , [10] were also observed in vivo ( Supplementary Fig. S3 ). 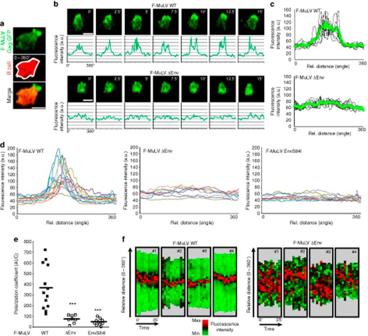Figure 2: Immobile F-MuLV-infected B cells polarize Gag-GFP in an Env glycoprotein-dependent manner. (a) Line profiles (0–360°) along the surface of B cells (red) resulted in fluorescence intensity profiles of surface Gag-GFP (green). Scale bar, 10 μm. (b) Gag-GFP (green) intensity line profiles over the interval of 15 min (every 2.5 min) of B cells infected with F-MuLV Gag-GFP expressing WT Env or lacking Env (ΔEnv;Supplementary Movies 3and4). Scale bar, 10 μm. (c) Average Gag-GFP intensity line profiles (green) for the two static cells shown inb. (d) Comparison of average Gag-GFP line profiles of various B cells infected with F-MuLV Gag-GFP WT (n=13), F-MuLV Gag-GFP ΔEnv (n=8) and F-MuLV Gag-GFP EnvS84I (n=10). (e) Gag-GFP polarization coefficient (Supplementary Fig. S2) of B cells infected with F-MuLV Gag-GFP WT, F-MuLV Gag-GFP ΔEnv or F-MuLV Gag-GFP EnvS84I for all events analysed ind. F-MuLV WT compared with ΔEnv: ***P=0.0002; F-MuLV WT compared with EnvS84I: ***P<0.0001 (Mann–Whitney test). (f) Polarization kymograph presentation of Gag-GFP fluorescence profiles (0–360°) over a time of 25 min for B cells infected with F-MuLV Gag-GFP containing WT Env or lacking Env (ΔEnv). Maximum 5% fluorescent intensity is displayed as red, minimum intensity as green. Figure 2: Immobile F-MuLV-infected B cells polarize Gag-GFP in an Env glycoprotein-dependent manner. ( a ) Line profiles (0–360°) along the surface of B cells (red) resulted in fluorescence intensity profiles of surface Gag-GFP (green). Scale bar, 10 μm. ( b ) Gag-GFP (green) intensity line profiles over the interval of 15 min (every 2.5 min) of B cells infected with F-MuLV Gag-GFP expressing WT Env or lacking Env (ΔEnv; Supplementary Movies 3 and 4 ). Scale bar, 10 μm. ( c ) Average Gag-GFP intensity line profiles (green) for the two static cells shown in b . ( d ) Comparison of average Gag-GFP line profiles of various B cells infected with F-MuLV Gag-GFP WT ( n =13), F-MuLV Gag-GFP ΔEnv ( n =8) and F-MuLV Gag-GFP EnvS84I ( n =10). ( e ) Gag-GFP polarization coefficient ( Supplementary Fig. S2 ) of B cells infected with F-MuLV Gag-GFP WT, F-MuLV Gag-GFP ΔEnv or F-MuLV Gag-GFP EnvS84I for all events analysed in d . F-MuLV WT compared with ΔEnv: *** P =0.0002; F-MuLV WT compared with EnvS84I: *** P <0.0001 (Mann–Whitney test). ( f ) Polarization kymograph presentation of Gag-GFP fluorescence profiles (0–360°) over a time of 25 min for B cells infected with F-MuLV Gag-GFP containing WT Env or lacking Env (ΔEnv). Maximum 5% fluorescent intensity is displayed as red, minimum intensity as green. Full size image Infected B cells form functional virological synapses in vitro The Env-dependent polarization of Gag in infected B cells in vivo is likely the consequence of the formation of a cell–cell interface with an unlabelled endogenous leucocyte within the popliteal lymph node. To confirm the ability of F-MuLV-infected B cells to form virological synapses and to identify the target cell type, we developed an ex vivo co-culture assay. Primary B cells infected with F-MuLV Gag-GFP/Env-mCherry were co-cultured with total leucocytes isolated from popliteal and inguinal lymph nodes of cytoplasmic GFP-expressing mice. Spinning-disc confocal microscopy revealed the formation of virological synapses defined by a concentration of F-MuLV Env and Gag in button or ring-like structures in the cell–cell interface and an orientation of the trans-Golgi network towards the cell–cell contact ( Fig. 3a , Supplementary Fig. S4 , Supplementary Movie 5 ). We used antibodies against various leucocyte surface markers to identify the target cells ( Supplementary Fig. S5 ). F-MuLV-infected B lymphocytes formed virological synapses predominantly with CD4 + T cells (70%) and CD19 + B cells (30%), but only infrequently with CD8 + T cells (14%; Fig. 3b ). As CD4 + T cells and CD8 + T cells were equally abundant in popliteal and inguinal lymph nodes of GFP-expressing mice ( Supplementary Fig. S6 ), we observed a more than threefold selectivity of virological synapses for CD4 + T cells over CD8 + T cells ( Fig. 3c ). The high motility of T cells in these co-cultures did not permit a precise capture of virus transfer from cell-to-cell using time-lapse video microscopy. We therefore co-cultured infected F-MuLV-infected B cells with adherent XC rat fibroblasts expressing mCAT-1-mCherrry where the transfer of GFP-positive punctae from infected B cells to target cells was readily detectable ( Fig. 3d , Supplementary Fig. S7 , Supplementary Movies 6 and 7 ). To test whether these cell–cell interactions also result in viral spread in vivo , we s.c. transferred in vitro -infected RFP-expressing B cells into the footpad of C57BL/6 mice and measured the Env-dependent viral spread to recipient leucocytes ( Fig. 3e ). Antibody staining of new infected leucocytes confirmed the selectivity of viral transfer to CD4 + T cells and not to CD8 + T cells in vivo ( Fig. 3g ). The increased spreading of F-MuLV to B cells observed in vivo ( Fig. 3g ) likely reflects the spatial organization of lymph nodes and the localization of the adoptively transferred F-MuLV-infected B cells to the B cell zone. Virological synapse formation between B cells was also occasionally observed in vivo by intravital microscopy after adoptive transfer of F-MuLV-infected cells expressing Gag-GFP (red/green) and uninfected B cells (red; Supplementary Fig. S8 , Supplementary Movie 8 ). 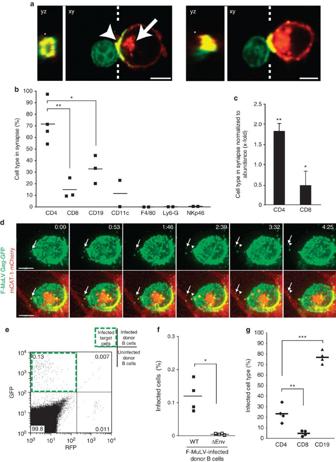Figure 3: F-MuLV-infected B cells form virological synapsesex vivowith CD4+T cells and B cells. (a) Confocal microscopy images of virological synapses between F-MuLV-infected B cells expressing Gag-GFP (green) and Env-mCherry (red) and total leucocytes (green) isolated from GFP-expressing transgenic mice. Images represent xy and yz images of a z-stack acquired from a fixedex vivoco-culture. yz orientation of images reveal ring- and button-shaped virological synapses (star) characterized by an accumulation of Gag-GFP (green) and Env-mCherry (red) at the cell–cell interface (arrowhead). The arrow depicts Env-mCherry-enriched trans-Golgi network polarizing towards the virological synapse. Scale bar, 5 μm. (b) Antibody staining against various leucocyte surface markers identifies CD4+T cells and CD19+B cells as target cells in virological synapses with F-MuLV-infected B cells. Data represent two to four independent experiments. CD4 compared with CD8: **P=0.0038, CD4 compared with CD19: *P=0.0181 (unpairedt-test). (c) Fold enrichment of cell types found in virological synapses with F-MuLV-infected B lymphocytesin vitrofrombnormalized to abundance in pooled popliteal and inguinal lymph nodes (Supplementary Fig. S6). Data are the mean±s.d. of three to four independent experiments. **P=0.0041, *P=0.0354 (unpairedt-test). (d) Cell–cell transfer of viral particles (Gag-GFP) from F-MuLV Gag-GFP-infected primary B cells to mCAT-1-mCherry-expressing XC cells over sites of cell–cell contacts. Images were taken at indicated intervals. Arrows and arrow heads depict site of particle transfer. Scale bar, 3 μm. (e) Flow cytometry analysis of the draining popliteal lymph node 6 days after s.c. transfer of F-MuLV-LTR-GFP-infected RFP-expressing B cells. RFP-positive cells were excluded by gating the RFP-negative cell population to specifically monitor viral spreading to cells from the recipient mouse (green rectangle). Numbers indicate the percentage to total leucocytes. (f) Frequency of F-MuLV-infected GFP-expressing leukocytes in draining popliteal lymph nodes 6 days after transfer of F-MuLV-LTR-GFP WT- and ΔEnv-infected B lymphocytes. *P=0.0286 (Mann–Whitney test). (g) Surface marker analysis of GFP-positive F-MuLV-infected cells of the popliteal lymph nodes frome. CD4 compared with CD8: **P=0.0032; CD4 compared with CD19: ***P<0.0001 (unpairedt-test). Figure 3: F-MuLV-infected B cells form virological synapses ex vivo with CD4 + T cells and B cells. ( a ) Confocal microscopy images of virological synapses between F-MuLV-infected B cells expressing Gag-GFP (green) and Env-mCherry (red) and total leucocytes (green) isolated from GFP-expressing transgenic mice. Images represent xy and yz images of a z-stack acquired from a fixed ex vivo co-culture. yz orientation of images reveal ring- and button-shaped virological synapses (star) characterized by an accumulation of Gag-GFP (green) and Env-mCherry (red) at the cell–cell interface (arrowhead). The arrow depicts Env-mCherry-enriched trans-Golgi network polarizing towards the virological synapse. Scale bar, 5 μm. ( b ) Antibody staining against various leucocyte surface markers identifies CD4 + T cells and CD19 + B cells as target cells in virological synapses with F-MuLV-infected B cells. Data represent two to four independent experiments. CD4 compared with CD8: ** P =0.0038, CD4 compared with CD19: * P =0.0181 (unpaired t -test). ( c ) Fold enrichment of cell types found in virological synapses with F-MuLV-infected B lymphocytes in vitro from b normalized to abundance in pooled popliteal and inguinal lymph nodes ( Supplementary Fig. S6 ). Data are the mean±s.d. of three to four independent experiments. ** P =0.0041, * P =0.0354 (unpaired t -test). ( d ) Cell–cell transfer of viral particles (Gag-GFP) from F-MuLV Gag-GFP-infected primary B cells to mCAT-1-mCherry-expressing XC cells over sites of cell–cell contacts. Images were taken at indicated intervals. Arrows and arrow heads depict site of particle transfer. Scale bar, 3 μm. ( e ) Flow cytometry analysis of the draining popliteal lymph node 6 days after s.c. transfer of F-MuLV-LTR-GFP-infected RFP-expressing B cells. RFP-positive cells were excluded by gating the RFP-negative cell population to specifically monitor viral spreading to cells from the recipient mouse (green rectangle). Numbers indicate the percentage to total leucocytes. ( f ) Frequency of F-MuLV-infected GFP-expressing leukocytes in draining popliteal lymph nodes 6 days after transfer of F-MuLV-LTR-GFP WT- and ΔEnv-infected B lymphocytes. * P =0.0286 (Mann–Whitney test). ( g ) Surface marker analysis of GFP-positive F-MuLV-infected cells of the popliteal lymph nodes from e . CD4 compared with CD8: ** P =0.0032; CD4 compared with CD19: *** P <0.0001 (unpaired t -test). Full size image F-MuLV infects B cells and CD4 + T cells in vivo MLV can be transmitted in mice by skin injury between fighting and biting adult mice in addition to the transfer from mother to offspring [13] , [15] . As we have studied F-MuLV spreading in the popliteal lymph node, we chose the skin route of transmission and s.c. delivered F-MuLV into the leg within the draining area of the popliteal lymph node. Adult mice were infected s.c. into the footpad with F-MuLV carrying a long terminal repeat (LTR)-GFP reporter that allowed for analysis of initially infected leucocytes ( Fig. 4a ). Flow cytometry after 2.5 days revealed that leucocytes in the draining popliteal lymph node were preferentially infected over those in other lymphoid organs, the inguinal lymph node and the spleen ( Fig. 4b ). Antibody staining for various leucocytes identified these cells as CD4 + T cells (~50%) and CD19 + B cells (~45%; Fig. 4c ; Supplementary Fig. S9 ). In a second experiment, we allowed for spread of the LTR-GFP reporter by infecting with replication-competent F-MuLV that can co-package and spread the reporter. These experiments revealed that at day 5, the infection of leucocytes in the popliteal lymph node had tripled in an Env-dependent manner while the ratio of infected cells had changed to ~30% infected T cells and ~60% infected B cells ( Fig. 4e ). Importantly, mice lacking B cells were resistant to early F-MuLV infection, demonstrating that the initial infection of CD4 + T cells was entirely dependent on the presence of B cells ( Fig. 4e ). We also determined the in vitro susceptibility of CD4 + and CD8 + T cells to F-MuLV infection and found that CD4 + and CD8 + T cells were equally susceptible to cell-free virus ( Fig. 4g ). In striking contrast, in the morphological context of the lymph node where F-MuLV-infected B cells were observed to form virological synapses ( Figs 1 and 2 ), the infection specifically spread to CD4 + T cells but not to CD8 + T cells ( Fig. 4f ). Thus, the ability of F-MuLV-infected B cells to form virological synapses with CD4 + T cells and B cells in vitro correlated with the spread of F-MuLV in vivo . 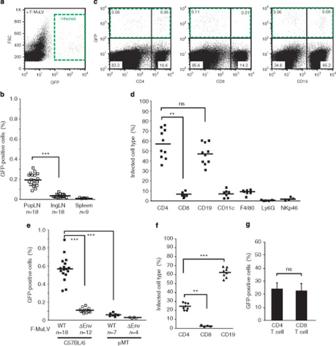Figure 4: F-MuLV infects B cells and CD4+T cellsin vivo. (a) Flow cytometry analysis of total popliteal leucocytes 2.5 days after s.c. infection of C57BL/6 mice with the reporter virus F-MuLV-LTR-GFP. (b) Frequency of F-MuLV-infected leucocytes in various lymph organs (popliteal lymph node, inguinal lymph node, spleen) 2.5 days after s.c. infection. ***P<0.0001 (Mann–Whitney test).nrepresents the number of analysed lymph nodes and spleens. (c) Flow cytometry analysis of leucocytes from a draining popliteal lymph node 2.5 days after s.c. injection of F-MuLV-LTR-GFP. Cells were stained with antibodies against CD4, CD8 and CD19 and cells were analysed for GFP expression and surface marker distribution. Green rectangles highlight F-MuLV-infected GFP-expressing cells. Numbers in each square represent percentage to total cells counted. (d) Surface marker analysis of F-MuLV-infected cells of the popliteal lymph node. ns (non-significant)P=0.0959; **P=0.002 (Mann–Whitney test). (e) Flow cytometry analysis of total popliteal leucocytes for GFP-positive cells 5 days after s.c. injection of F-MuLV-LTR-GFP in the presence of full-length F-MuLV expressing Env (WT) or lacking Env (ΔEnv) into C57BL/6 mice or B cell-deficient μMT mice. C57BL/6 WT compared with ΔEnv: ***P<0.0001; C57BL/6 WT compared with μMT WT: ***P=0.0006 (Mann–Whitney test).nrepresents the number of analysed lymph nodes. (f) Analysis of F-MuLV-infected GFP-positive cells of the popliteal lymph node of C57BL/6 mice using antibodies against CD4, CD8 and CD19. CD4 compared with CD8: **P=0.0022, CD4 compared with CD19: ***P=0.0009 (Mann–Whitney test). (g)In vitrotransduction of primary CD4+and CD8+T cells with cell-free F-MuLV-LTR-GFP. Percentage of infected GFP-positive cells 24 h after infection. Data are the mean±s.d. of three independent experiments. ns (nonsignificant)P=0.4 (Mann–Whitney test). Figure 4: F-MuLV infects B cells and CD4 + T cells in vivo . ( a ) Flow cytometry analysis of total popliteal leucocytes 2.5 days after s.c. infection of C57BL/6 mice with the reporter virus F-MuLV-LTR-GFP. ( b ) Frequency of F-MuLV-infected leucocytes in various lymph organs (popliteal lymph node, inguinal lymph node, spleen) 2.5 days after s.c. infection. *** P <0.0001 (Mann–Whitney test). n represents the number of analysed lymph nodes and spleens. ( c ) Flow cytometry analysis of leucocytes from a draining popliteal lymph node 2.5 days after s.c. injection of F-MuLV-LTR-GFP. Cells were stained with antibodies against CD4, CD8 and CD19 and cells were analysed for GFP expression and surface marker distribution. Green rectangles highlight F-MuLV-infected GFP-expressing cells. Numbers in each square represent percentage to total cells counted. ( d ) Surface marker analysis of F-MuLV-infected cells of the popliteal lymph node. ns (non-significant) P =0.0959; ** P =0.002 (Mann–Whitney test). ( e ) Flow cytometry analysis of total popliteal leucocytes for GFP-positive cells 5 days after s.c. injection of F-MuLV-LTR-GFP in the presence of full-length F-MuLV expressing Env (WT) or lacking Env (ΔEnv) into C57BL/6 mice or B cell-deficient μMT mice. C57BL/6 WT compared with ΔEnv: *** P <0.0001; C57BL/6 WT compared with μMT WT: *** P =0.0006 (Mann–Whitney test). n represents the number of analysed lymph nodes. ( f ) Analysis of F-MuLV-infected GFP-positive cells of the popliteal lymph node of C57BL/6 mice using antibodies against CD4, CD8 and CD19. CD4 compared with CD8: ** P =0.0022, CD4 compared with CD19: *** P =0.0009 (Mann–Whitney test). ( g ) In vitro transduction of primary CD4 + and CD8 + T cells with cell-free F-MuLV-LTR-GFP. Percentage of infected GFP-positive cells 24 h after infection. Data are the mean±s.d. of three independent experiments. ns (nonsignificant) P =0.4 (Mann–Whitney test). Full size image Our understanding of retrovirus spreading is critically influenced by the concept of virological synapses that explains efficient virus cell-to-cell transmission via long-lived cell–cell interfaces between infected and uninfected cells [1] , [2] , [3] , [16] . Here we identify such Env-dependent long-lived contacts that polarize viral capsid towards the cell–cell interface between a subpopulation of F-MuLV-infected B cells and uninfected leucocytes in vivo . Using an in vitro co-culture assay, we identify the target cells as CD4 + T cells and CD19 + B cells. As the ability of infected B cells to form virological synapses with these cell types correlated with the viral spread in vivo , our results suggest that virological synapses can contribute to viral spreading in living mice. Although our data validate the concept of long-lived virological synapses in vivo , they do not exclude the possibility that cell-free virus or migratory leucocytes also contribute to viral spreading by more transient cell–cell interactions. Short-lived and more dynamic motile kinapses have also been observed in vivo studying immunological synapses [17] , [18] . Further improving intravital imaging technologies will permit the capture of virus transmission events during more transient cell–cell interactions. Our intravital imaging approach revealed a critical role for B cells during early MuLV infections. B cells also have important roles in the viral spread and in the pathogenesis of other retroviruses such as human T-cell lymphotropic virus type 1 and the mouse mammary tumour virus [19] , [20] . Although we demonstrate that B cells are early targets during F-MuLV infections, they also have a critical role in the development of an adaptive immune response. Antibody-mediated response together with a cytotoxic CD8 + T cell response will ultimately control F-MuLV infections in adult mice [21] , [22] . Antigen presentation by specialized immune cells induces adaptive immune responses. The here described polarized cell–cell contacts of F-MuLV-infected B cells, however, do not function as antigen presentation by B cells. A single point mutation in the receptor-binding domain of F-MuLV (S84I) that lowers the affinity for the viral receptor mCAT-1 (refs 4 , 23 ) completely abrogates the formation of stable contacts. This characterizes these interactions as virological synapses that are the consequence of Env–receptor interactions and distinguishes them from phenotypically similar immunological synapses. In vivo virological synapses, while resembling in many aspects their in vitro observed counterparts, show one striking difference. In vitro , synapse formation for F-MuLV is entirely driven by Env–receptor interactions [4] , [8] . In contrast, in vivo as well as in co-cultures with primary cells, F-MuLV-infected primary B cells selectively interact with CD4 + T cells and less with CD8 + T cells despite the fact that both cell types express similar mCAT-1 receptor levels and are equally susceptible to cell-free F-MuLV. Other factors in addition to the interaction of Env and receptor must therefore contribute to the selectivity of F-MuLV spreading in vivo . Thus, applying intravital imaging to monitor retroviral spreading directly in living mice provides insights into early infection events and viral spread of F-MuLV and establishes intravital imaging as a tool to monitor viral spreading directly in living animals. During the review of this manuscript, a related paper was published by Murooka et al . [24] Intravital imaging of HIV-infected migrating T cells in humanized mice confirmed a role of the viral glycoprotein in adhesive interactions with uninfected cells. Thus, both studies verify some of the main concepts of the virological synapses in vivo and suggest that transient interactions of migrating lymphocytes as well as long-lived virological synapses can contribute to retroviral spread in living organisms. Mice C57BL/6 mice were purchased from Harlan. Strains of mice expressing cytoplasmic RFP in all nucleated cells under control of the β-actin promoter (Tg(CAG-DsRed*MST)1Nagy/J) or cytoplasmic GFP via the ubiquitin promoter (Tg(UBC-GFP)30Scha/J) were obtained from Jackson Laboratory. B cell-deficient μMT mice (B6.129S2-Ighmtm1Cgn/J) were obtained from Jackson Laboratory. All experiments were approved by the Yale University Institutional Animal Care and Use Committee and Yale Institutional Biosafety Committee. Virus plasmids and virus preparation F-MuLV viral constructs generating Gag-GFP-labelled virions in primary cells were described previously [25] . Briefly, these viruses were generated in HEK293 cells by transfection of a pLRB303 plasmid encoding full-length F-MuLV [26] , [27] that carried a GFP protein fused to the carboxy terminus of Gag at the position of Pol and a plasmid encoding F-MuLV GagPol to compensate for the absence of Pol. When these viruses infect primary cells, they will generate and disseminate Gag-GFP-labelled particles, but due to the absence of Pol in the viral genome they will not be replication competent. F-MuLV viral constructs lacking Env were generated using the same pLRB303 plasmid encoding Gag-GFP and carrying two premature stop codons in Env as well as the additional presence of F-MuLV GagPol and a pcDNA3 plasmid encoding F-MuLV Env [4] . F-MuLV viral constructs with EnvS84I were generated by PCR leading to a serine to isoleucine substitution at position 84 of F-MuLV Env as described in Davey et al . [23] F-MuLV virus preparation expressing Gag-GFP- and Env-mCherry-labelled virions were generated by transfection of a pLRB303-derived plasmid encoding F-MuLV Gag-GFP and a mCherry insertion into the position 273 of Env as described previously [28] and the additional presence of F-MuLV GagPol and the pcDNA3 plasmid encoding F-MuLV Env. All F-MuLV preparations were generated in HEK293 cells cultured in 10 cm dishes with RPMI/10% fetal bovine serum/10 mM HEPES and transfected with 12 μg of total plasmid DNA using Fugene6 transfection reagent (Promega). After 24 and 48 h, cell supernatant was filtered using a 0.45 μm nylon membrane filter and stored at −80 °C. Primary cell culture Primary mouse T cells (CD4 + and CD8 + ) and B cells were isolated from splenocytes of C57BL/6 mice or mice ubiquitously expressing RFP using the EasySep Negative Selection Mouse T- or B Cell Enrichment Kits (StemCell Technologies), respectively. Primary cells were cultured in RPMI/10% fetal bovine serum supplemented with 10 mM HEPES, 1/100 non-essential amino acids (Gibco), 1 mM sodium pyruvate and 2 μM β-mercaptoethanol. CD4 + and CD8 + T lymphocytes were cultured in 96-well round-bottom tissue culture plates in the presence of recombinant mouse interleukin (IL)-7 (100 units ml −1 ) and IL-15 (100 units ml −1 ) and activated with phorbol myristate acetate (10 nM) and ionomycin (0.4 μM). Primary B lymphocytes were cultured in 96 well flat-bottom plates supplemented with recombinant mouse IL-4 (10 units ml −1 ) and IL-15 (100 units ml −1 ). B cells were activated using 7.5 μg ml −1 lipopolysaccharide from Escherichia coli (Invivogen). For in vitro transduction of activated primary mouse lymphocytes, concentrated virus was spinoculated onto 1.25 × 10 6 cells in the presence of polybrene (7.5 μg ml −1 ). Cells were trypsinized 8–12 h post infection to remove residual virus. Intravital microscopy and image analysis To visualize retrovirus-infected lymphocytes in vivo , we monitored the popliteal lymph nodes of anesthetized mice. Around 18–20 h post in vitro infection with F-MuLV Gag-GFP lymphocytes were adoptively transferred to 8–12-week-old C57BL/6 mice by s.c. injection into the footpad of the right limb. Cells were monitored 16–24 h after transfer by intravital microscopy. Mice were initially anesthetized by intraperitoneal injection of a ketamine and xylazine mixture and subsequently with nebulized isoflurane/O 2 gas mixture. Animals were immobilized on a custom-built stage and the right popliteal lymph node was surgically prepared. The lymph node was immersed in saline and covered with a glass coverslip. Temperature of the lymph node was maintained at 37 °C during imaging. Intravital microscopy of B cells confirmed proper homing into B cell follicles within the popliteal lymph node ( Supplementary Movie 2 ). For image acquisition, an Olympus BX51WI fluorescence microscope with a 20 × , 1.00 NA water immersion Zeiss objective and dedicated single-beam LaVision TriM Scope II (LaVision Biotec) was controlled by Imspector software. The microscope was outfitted with a Chameleon Vision II Ti:Sapphire laser (Coherent) with pulse precompensation. Emission wavelengths were collected with two photomultiplier tubes (Hamamatsu) for 412–472 nm (cyan fluorescent protein, CFP, second harmonic signal) and for 567–647 nm (RFP), respectively, and a GaAsP detector (Hamamatsu) for emission wavelengths of 500–550 nm (GFP). For four-dimensional (4D) analysis of cell migration, stacks of 21 optical sections with 3 μm z-spacing were acquired every 30 s for 30–60 min with the laser tuned to a wavelength of 900 nm. Each xy plane spanned 512 pixels each dimension with a resolution of 0.779 μm per pixel. Volocity software (PerkinElmer) was used for 4D tracking of individual cells. All cell tracks were individually examined to confirm that they reported the behaviour of a single cell. Volocity and ImageJ were used to create QuickTime-formatted movies of image sequences. Fluorescent intensity line profiles were generated with Volocity software by drawing a 1-μm-thick line around cell surface (cytoplasmic RFP) of the z-plane of a stack representing the cell centre. Fluorescence intensity profiles and heat maps were analysed and generated using Microsoft Excel. The polarization coefficient of virological synapses in vivo was analysed using the average fluorescence Gag-GFP line profile over time. The trendline for fluorescent values above mean intensity of each synapse was determined using Microsoft Excel. The area below the polygonal best fit trendline (area under the curve) of each average polarization line profile was determined by integration. The area under the curve is used as a measure for extent of polarization ( Supplementary Fig. S2 ). F-MuLV infection in vivo For reporter virus production, HEK293 cells were co-transfected with pLRB303-derived plasmid encoding full-length F-MuLV +Env or −Env and the additional plasmid pMMP-LTR-GFP expressing cytoplasmic GFP (1/10) [29] . Viral titre was determined by titrating concentrated virus on the murine T-lymphoid S49.1 cell line. GFP expression was determined after 24 h using flow cytometry. For in vivo studies using cell-free virus 1.5–4 × 10 5 infectious, F-MuLV units were s.c. transferred into C57BL/6 mice or B cell-deficient μMT mice. For in vivo studies using F-MuLV-infected lymphocytes, RFP-expressing B cells were transduced in vitro with F-MuLV-LTR-GFP and transferred into the footpad of C57BL/6 mice. Viral spreading was quantified after 6 days by analysing RFP-negative leucocytes. Characterization of F-MuLV-infected leucocytes was done by flow cytometry for GFP-expressing cells using FACSCanto (BD). After indicated time points post infection single-cell suspension from lymph nodes (popliteal and inguinal) and spleen were prepared. Lymph nodes were incubated for 20 min at 37 °C with Liberase TL (0.2 mg ml −1 ) and DNase I (20 μg ml −1 ) followed by passing the tissue through a 70 μm cell strainer. Red blood cell lysis was performed with splenocytes. For immunostaining, cell suspensions were fixed with 4% PFA and subsequently incubated with antibodies against various surface markers. Data were analysed with FlowJo software (Tree Star). Flow cytometry antibodies The following antibodies were used: GpCD4 (clone RM4-5, BioLegend), CD8a (clone 53-6.7, BioLegend), CD19 (clone 1D3, BD) or CD11c-allophycocyanin (clone N418, BD), anti-F4/80 (clone CI:A3-1), anti-NKp46 (clone 29A1.4) and anti-Ly-6G (clone 1A8). An allophycocyanin-conjugated goat antibody against rat immunoglobulin G (BioLegend) was used as secondary antibody. In vitro co-culture assay To analyse virological synapse formation in vitro , a co-culture system with MLV-infected B lymphocytes and total leucocytes was developed. To support physiological migration of naive leucocytes on two-dimensional surface, glass-bottom cover slips were coated over night with 8 μg ml −1 intercellular adhesion molecule 1 and 2.5 μg ml −1 chemokine (C-C motif) ligand 21. To visualize virological synapses and to identify target cell types, activated B lymphocytes were infected with F-MuLV encoding Gag-GFP and Env–mCherry fusion proteins within the context of the full-length genome. Residual virus was removed 12 h after spinoculation by trypsin treatment. Around 18 h post infection, MLV-infected B cells were co-cultured (ratio 1:2) with leucocytes from inguinal and popliteal lymph nodes of cytoplasmic GFP-expressing mice. Co-culture was incubated for 12–18 h before fixation with 4% PFA. To identify target cell types, fixed samples were immunostained for leucocyte surface markers. The following antibodies (BioLegend) were used: anti-CD3 (clone 17A2), anti-CD4 (clone RM4-5, BioLegend), anti-CD8a (clone 53-6.7), anti-CD19 (clone 1D3), anti-CD11c (clone N418), anti-F4/80 (clone CI:A3-1), anti-NKp46 (clone 29A1.4) and anti-Ly-6G (clone 1A8). As secondary antibodies anti-rat/-hamster-Alexa568 (Invitrogen) were used and samples were embedded in ProLong-Gold antifade reagent (Invitrogen). To visualize transfer of viral particles by 4D microscopy, B lymphocytes isolated from C57BL/6 mice were infected with F-MuLV Gag-GFP before co-culture with rat XC sarcoma cells [30] expressing mCAT-1-mCherry. Images were acquired using a Nikon spinning-disc confocal microscope and analysed using the Volocity software (PerkinElmer). Statistical analysis For statistical analysis, data were analysed by unpaired t -test or Mann–Whitney test as stated in each case and the P -value was calculated. How to cite this article: Sewald, X. et al . In vivo imaging of virological synapses. Nat. Commun. 3:1320 doi: 10.1038/ncomms2338 (2012).